Three decades of high-resolution coastal sea surface temperatures reveal more than warming Understanding and forecasting current and future consequences of coastal warming require a fine-scale assessment of the near-shore temperature changes. Here we show that despite the fact that 71% of the world's coastlines are significantly warming, rates of change have been highly heterogeneous both spatially and seasonally. We demonstrate that 46% of the coastlines have experienced a significant decrease in the frequency of extremely cold events, while extremely hot days are becoming more common in 38% of the area. Also, we show that the onset of the warm season is significantly advancing earlier in the year in 36% of the temperate coastal regions. More importantly, it is now possible to analyse local patterns within the global context, which is useful for a broad array of scientific fields, policy makers and general public. Coastal marine ecosystems yield nearly half of the Earth's total ecosystem goods and services [1] . Simultaneously, coastal ecosystems are among the most highly impacted marine systems [2] , suffering from the cumulative pressure of anthropogenic land-based processes such as overpopulation, agricultural runoff and pollution, and also ocean-based human activities like overfishing and intense maritime traffic [2] , [3] . Superimposed on such local factors are those associated with climate change, which have the added potential to exacerbate other anthropogenic effects [4] . The recent change in sea temperature is considered as the most pervasive and severe cause of impact in coastal ecosystems worldwide [2] . Although multiple climatological studies have shown that both land surface and sea surface temperatures (SSTs) have been generally increasing since the beginning of the instrumental record [5] , [6] , [7] , [8] , higher-resolution studies are still needed. For instance, spatial or temporal data binning, a common way to deal with data scarcity, may result in artificial a priori clustering and therefore conceal the position of data discontinuities or inflexion points, especially when performed at large scales. Also, most global warming assessment studies lack information on the seasonality of such changes. It is hence undeniable that a broad range of scientific disciplines, in addition to resource managers, policy makers and even the general public, would benefit by having finer-scale data. Still, advances in this area have been hindered by the lack of global, accurate, high-resolution observations obtained by means of standardized methods [7] . Recently, National Oceanic and Atmospheric Administration (NOAA) has released a spatially complete SST product offering unparalleled temporal coverage and temporal and spatial resolution (Optimum Interpolation (OI) ¼ Degree Daily SST Analysis [9] data, also known as Reynolds 0.25 v.2). Even though limited to the last three decades, the data set encompasses the recent period of strongest global warming [5] , [6] allowing for a detailed analysis of the warming processes and patterns since the early 1980s. Here we present quantitative estimates of changes in coastal SST with unprecedented levels of spatial and temporal resolution worldwide. First, we explore global and monthly warming patterns along the world's coastlines at a scale of 0.25° for the last three decades. Second, we quantify the changes in the yearly frequency of extremely cold and extremely warm events. Finally, given the influence that seasonal temperature fluctuations have in driving phenological changes [10] , [11] , [12] , [13] , we quantify the observed changes in the timing of seasonal warming. Global patterns In total, 19,276 coastal locations were analysed, corresponding to an area exceeding 9×10 6 km 2 (for detailed analyses for each location separately, refer to Supplementary Data 1 , or to www.coastalwarming.com ). In the last three decades, ∼ 71.6% of this area experienced significant ( P <0.05) increases in SST, at a mean rate of 0.25±0.13 °C per decade (mean±s.e.m. ), see Fig. 1a . There has been significant ( P <0.05) cooling in 6.8% of the area (−0.11±0.10 °C per decade in average). In the remaining 22.2% of the coast, no significant changes were detected. In agreement with previous studies [6] , [7] , [8] , higher coastal warming rates were observed between the Tropic of Cancer and the Arctic Circle, especially along the margins of enclosed or semienclosed seas or in narrow areas with complex coastal morphology. This included most of the Eurasian and North American seas, bays and gulfs ( Fig. 2a ). Nonetheless, intense warming rates were also observed in open coasts such as off Eastern China, Western Africa or Northeast South-America. Significant decreases in SST were registered mainly at middle latitude portions of the Southwestern and Eastern US coasts, Western South-America and Western Australia. 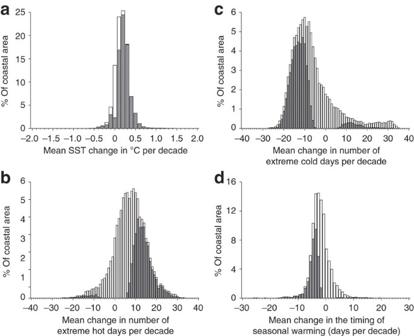Figure 1: Frequency histograms for percentage change of coastal area. While white bars represent all data, grey bars show only data from locations in which rates of change were statistically significant. (a) Percentages of coastal area and respective SST changes in °C per decade. (b) percentages of coastal area and respective rates of change in the yearly frequency of extreme hot events, in number of days per decade. (c) Percentages of coastal area and respective rates of change in the yearly frequency of extreme cold events, in number of days per decade. (d) Percentages of coastal area with different rates of change in the timing of seasonal warming, in number of days per decade. The bin size inais 0.1 °C and inb,canddis 1 day. Figure 1: Frequency histograms for percentage change of coastal area. While white bars represent all data, grey bars show only data from locations in which rates of change were statistically significant. ( a ) Percentages of coastal area and respective SST changes in °C per decade. ( b ) percentages of coastal area and respective rates of change in the yearly frequency of extreme hot events, in number of days per decade. ( c ) Percentages of coastal area and respective rates of change in the yearly frequency of extreme cold events, in number of days per decade. ( d ) Percentages of coastal area with different rates of change in the timing of seasonal warming, in number of days per decade. The bin size in a is 0.1 °C and in b , c and d is 1 day. 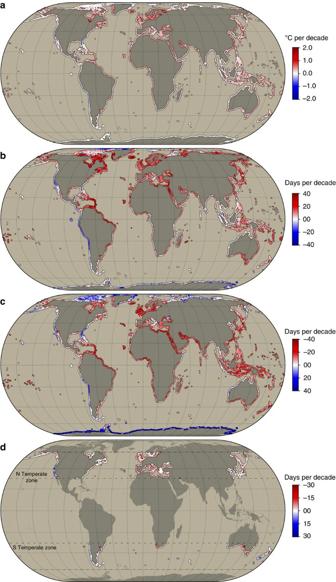Figure 2: Changes in temperature along the world's coastlines. (a) warming rates for the period between 1982 and 2010, expressed in °C per decade. Red indicates warming and blue indicates cooling. (b) Linear trends in the yearly frequency of extreme hot days, in number of days per decade. Red indicates increase and blue indicates decrease in the number of events. (c) Linear trends in the yearly frequency of extreme cold days, in number of days per decade. Red indicates decrease and blue indicates increase in the number of events. (d) Linear trends in the timing of seasonal warming for the temperate regions, expressed in number of days per decade. Red indicates an advance and blue indicates a delay in the timing of seasonal warming. Full size image Figure 2: Changes in temperature along the world's coastlines. ( a ) warming rates for the period between 1982 and 2010, expressed in °C per decade. Red indicates warming and blue indicates cooling. ( b ) Linear trends in the yearly frequency of extreme hot days, in number of days per decade. Red indicates increase and blue indicates decrease in the number of events. ( c ) Linear trends in the yearly frequency of extreme cold days, in number of days per decade. Red indicates decrease and blue indicates increase in the number of events. ( d ) Linear trends in the timing of seasonal warming for the temperate regions, expressed in number of days per decade. Red indicates an advance and blue indicates a delay in the timing of seasonal warming. Full size image The number of yearly extremely hot days has significantly ( P <0.05) increased in 38.1% of the world's coastal areas, at a mean rate of 13.8±6.4 days per decade ( Fig. 1b ). Only 1.2% of the world's coastlines witnessed a significant ( P <0.05) decrease in the number of yearly extremely hot days (at a mean rate of −12.9±6.0 days per decade). Changes in the number of extreme hot days were significantly correlated with the intensity of warming (Pearson's r =0.73, d.f.=964, P <0.01). Hence, regions that have been warming the most also tend to be experiencing an increase in the frequency of hot events (for example, North, Baltic and Mediterranean Seas, Eastern North-America, Eastern South-America, among other; compare Fig. 2a and b ). The coasts of Western North America, Western South-America and Antarctica showed the highest decreases in the frequency of extreme hot days. Changes in the number of yearly extreme cold days were negatively correlated with the rates of change of SST (Pearson's r =−0.70, d.f.=964, P <0.01). Extreme cold events have significantly ( P <0.05) decreased in 45.8% of the worlds' coastline, at a mean rate of 13.1±5.5 days per decade ( Fig. 1c ). Larger decreases have occurred off North West Europe, Northeast North-America, Northeast South-America, Western Mediterranean, North West Indian Ocean, Southeast Asia, South Australia and New Zealand ( Fig. 2c ). Conversely, extreme cold events have significantly ( P <0.05) increased in frequency only in 3% of the worlds' coastlines (particularly at very high latitudes in North Eurasia, North America and Antarctica, but also off the West South-America, Southeast and Western North-America and Western Australia), at a mean rate of 14.1±7.3 days per decade ( Fig. 2c ). In general, increases in extreme hot days were accompanied by decreases in extreme cold events (Pearson's r =−0.55, d.f.=964, P <0.01). A simultaneous increase in the frequency of hot extremes and decrease in cold extremes occurred in 74.8% of the coastlines, while in 10.4% of the area there was a simultaneous increase in the frequency of both temperature extremes. An example in northern Europe was 2009–2010 when one of the coldest winters of the past century [14] was followed by one of the hottest summers since the 1500s [15] . In 35.7% of the temperate coastal area (between latitudes 30° and 60° in both hemispheres), seasonal warming has been occurring significantly ( P <0.05) earlier in the year, at an average rate of 6.1±3.2 days per decade ( Fig. 1d ). This change in seasonal timing was also inversely correlated with the average change in SST (Pearson's r =−0.46, d.f.=251, P <0.01). Accordingly, the highest advances in the seasonal warming were observed off sheltered or semienclosed portions of the coast, particularly in the Northeast Atlantic and Mediterranean coasts, and also off South Africa and South Australia ( Fig. 2d ). Only 0.4% of the temperate area (mainly off Western North-America, Western South-America and Southwest New Zealand) witnessed a significant delay ( P <0.05) in seasonal warming (at a mean rate of 8.6±6.1 days per decade). Continental-scale latitudinal transects Along the Eastern Atlantic coast, SST has risen at a mean rate of 0.27.±0.13 °C per decade since 1982. Particularly rapid increases were observed along the margins of both the Norwegian and North Seas, at rates varying between ∼ 0.3 and ∼ 0.7 °C per decade. There is a wealth of information associating this warming with poleward shifts in species' geographical ranges, phenology changes to earlier dates in the year, and ecosystem regime changes from cold-water to warm-water assemblages [14] , [16] , [17] , [18] , [19] , [20] . SST has not been increasing homogeneously during the year, but rather changes have been more rapid during spring and autumn ( Fig. 3a ). Along the Southwest European coast, SST has been increasing from ∼ 0.2 to ∼ 0.3 °C per decade (mostly in summer). Also in this region, several poleward shifts in species' geographical ranges were associated with rising SST [14] , [21] , [22] . In Northwest Africa, in the region dominated by the Canary Current (northwards from Cap Blanc), warming rates have been more modest ( ∼ 0.1 to 0.2 °C per decade). At Cap Blanc (transition between areas 6–7, Fig. 3 ), the poleward North Equatorial Counter Current meets the Canary Current, forming a large oceanographic discontinuity [23] . That region has witnessed large rates of warming, especially during the summer. From there and towards the Gulf of Guinea (along the areas 6–8, Fig. 3 ), warming seasonality gradually inverted becoming stronger from October to April. Warming rates peaked again north of the Angola-Benguela front (transition between areas 9 and 10, Fig. 3 ), where the poleward Angola Current collides with the Benguela Current, which drifts offshore [23] . SST in this region increased up to ∼ 0.4 °C per decade, which has been related to major ecosystem shifts in the area [24] . Off Southwest Africa, temperatures have been decreasing slightly (particularly from January to May, Fig. 3a ). 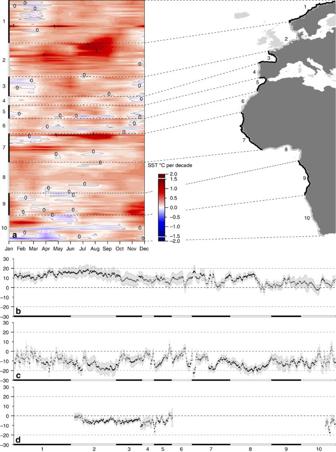Figure 3: Latitudinal transect along the Eastern Atlantic Ocean. (a) Linear rates of SST change along the Eastern Atlantic coast, expressed in °C per decade. Horizontal axis is month within the year and vertical axis represents location along the coastline. (b) Average change in the yearly frequency of extreme hot days, in days per decade. (c) Average change in the yearly frequency of extreme cold days, in days per decade. (d) Average change in the occurrence of seasonal warming, in days per decade. Inb,candd, significant data are depicted in black and nonsignificant in grey. Numbered black and white portions of the horizontal axis can be used to locate sections of the coastline in the geographical map. Confidence intervals represent s.e.m. Figure 3: Latitudinal transect along the Eastern Atlantic Ocean. ( a ) Linear rates of SST change along the Eastern Atlantic coast, expressed in °C per decade. Horizontal axis is month within the year and vertical axis represents location along the coastline. ( b ) Average change in the yearly frequency of extreme hot days, in days per decade. ( c ) Average change in the yearly frequency of extreme cold days, in days per decade. ( d ) Average change in the occurrence of seasonal warming, in days per decade. In b , c and d , significant data are depicted in black and nonsignificant in grey. Numbered black and white portions of the horizontal axis can be used to locate sections of the coastline in the geographical map. Confidence intervals represent s.e.m. Full size image In general, the frequency of extreme hot days has increased along the Eastern Atlantic margin by 8.4±6.6 additional hot days per decade in average ( Fig. 3b ). Such changes are particularly evident in the North Sea and English Channel and Northwest and central Africa. Extreme cold events, in contrast, have decreased in frequency at a mean rate of 11.2±7.1 days per decade, with most significant changes occurring in the North Sea, Bay of Biscay and off the Northwest and central African coast ( Fig. 3c ). Seasonal warming has been occurring earlier in most of the temperate Eastern Atlantic, at a mean rate of 5.6±4.3 days per decade. Off the North Sea, English Channel, Bay of Biscay and Northwest Africa (areas 2, 3 and 5, Fig. 3 ), most changes were significant. In the Northwest Atlantic, coastal SST rose the fastest at higher latitudes, exceeding 1.0 °C per decade in several portions of the Labrador Sea, the Gulf of St Lawrence and the Bay of Fundy, particularly during Spring and Autumn ( Fig. 4a ), which may be related with the weakening of the North Atlantic Subpolar Gyre [25] and the Labrador Current [26] . South from the Bay of Fundy, coastal waters have warmed in average at ∼ 0.1 to 0.3 °C per decade ( Fig. 2a ), mainly in the summer ( Fig. 4a ). Warming patterns off Northeast North-America were mirrored by changes in the number of extreme hot and extreme cold days ( Fig. 4b,c ). Seasonal warming also tended to occur earlier in the year (areas 2–5, Fig. 4d ). Interestingly, poleward range shifts have already been reported for intertidal species and pelagic fish communities in this region [27] , [28] . In region 6, south of Cape Hatteras, one of the areas with strongest cooling worldwide, temperature change has gone the opposite direction (between −1.0 and −2.0 °C per decade in January at some locations, Fig. 4a ). This cooling is consistent with previous reports [6] , [8] and may be linked to changes in the path of the Gulf Stream, especially in winter [29] . Along the remaining Western Atlantic, SST has been warming at rates between 0.1 and 0.2 °C per decade in the coasts of Gulf of Mexico, Eastern Brazil, South Argentina and Tierra del Fuego, while off North South-America, South Brazil, Uruguay and North Argentina, SST has warmed at faster rates, between 0.2 and 0.4 °C per decade ( Fig. 4a ). Warming has been homogeneous through the year along the entire East South-American continent ( Fig. 4a ). The number of extreme hot days has also increased significantly off Northeast South-America, exceeding 10 extra hot days per decade along large portions of the coast ( Fig. 4b ). This pattern was mirrored by the change in number of extreme cold days, with many locations showing symmetrical changes in the number of extreme cold days ( Fig. 4c ). The exceptional positive rates off Southeast United States (exceeding 10 extra cold days per decade) are also noteworthy. 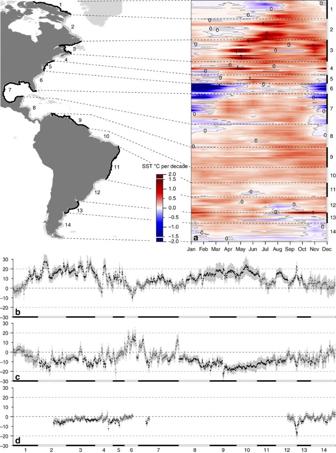Figure 4: Latitudinal transect along the Western Atlantic Ocean. (a) Linear trends of SST change along the Western Atlantic coast, expressed in °C per decade. Horizontal axis is month within the year and vertical axis represents location along the coastline. (b) Average change in the yearly frequency of extreme hot days, in days per decade. (c) Average change in the yearly frequency of extreme cold days, in days per decade. (d) Average change in the occurrence of seasonal warming, in days per decade. Inb,candd, significant data are depicted in black and nonsignificant in grey. Numbered black and white portions of the horizontal axis can be used to locate sections of the coastline in the geographical map. Confidence intervals represent s.e.m. Figure 4: Latitudinal transect along the Western Atlantic Ocean. ( a ) Linear trends of SST change along the Western Atlantic coast, expressed in °C per decade. Horizontal axis is month within the year and vertical axis represents location along the coastline. ( b ) Average change in the yearly frequency of extreme hot days, in days per decade. ( c ) Average change in the yearly frequency of extreme cold days, in days per decade. ( d ) Average change in the occurrence of seasonal warming, in days per decade. In b , c and d , significant data are depicted in black and nonsignificant in grey. Numbered black and white portions of the horizontal axis can be used to locate sections of the coastline in the geographical map. Confidence intervals represent s.e.m. Full size image SSTs have risen exceptionally rapidly off Northwest North-America during summer and autumn. On Western Alaska, for example, SST increases have exceeded 1.0 °C per decade around July ( Fig. 5a ), frequently in combination with an increase in the yearly frequency of extreme hot days ( Fig. 5b ). Along this coastline, changes in the number of extreme cold days varied from a few additional days per decade in sheltered stretches of the coast (fjords) to less than 10 cold days per decade at capes or open coast locations ( Fig. 5c ). In general, seasonal warming has been occurring significantly earlier ( Fig. 5d ). Further south, along Western Central-America and Northwest South-America, SST has also been increasing slightly, in particular around the months of April and September. In the Eastern Pacific lie two of the major coastal currents associated with upwelling areas, worldwide: the California Current (off Western United States, 4–5 in Fig. 5 ) and the Humboldt Current (off Chile and Peru, 8–9 in the same map) [30] . SST has decreased nearly year-round in the regions influenced by these currents (up to −0.4 °C per decade), in agreement with several studies describing a tendency for the intensification of the upwelling in the area [31] , [32] . Decreases in SST have been accompanied by lower frequencies of extreme hot days ( Fig. 5b ) and by a significant increase in the number of cold days ( Fig. 5c ). Although not strong enough to be significant, there is a tendency for a delay in the seasonal warming off California and Chile ( Fig. 5d ). Temperatures on these coasts are largely dominated by decadal changes in circulation patterns such as the Pacific Decadal Oscillation and the El Niño/Southern Oscillation [33] , [34] , which frequently alternate between contrasting warm and cold phases. Large-scale temperature fluctuations are important drivers on the biogeographic patterns observed on the Eastern pacific coast [35] , and while several studies have reported population and poleward range shifts associated with episodes of abnormally high SST [36] , [37] , others show that during cold phases species distributions may be driven in equatorialwards [33] , or may not change at all [38] . 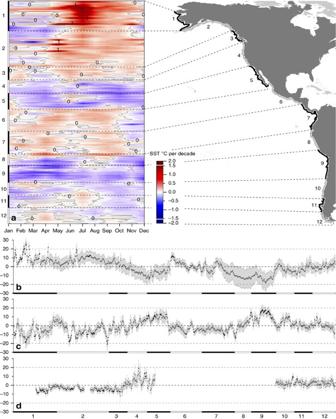Figure 5: Latitudinal transect along the Eastern Pacific Ocean. (a) Linear trends of SST change along the Eastern Pacific coast, expressed in °C per decade. Horizontal axis is month within the year and vertical axis represents location along the coastline. (b) Average change in the yearly frequency of extreme hot days, in days per decade. (c) Average change in the yearly frequency of extreme cold days, in days per decade. (d) Average change in the occurrence of seasonal warming, in days per decade. Inb,candd, significant data are depicted in black and nonsignificant in grey. Numbered black and white portions of the horizontal axis can be used to locate sections of the coastline in the geographical map. Confidence intervals represent s.e.m. Figure 5: Latitudinal transect along the Eastern Pacific Ocean. ( a ) Linear trends of SST change along the Eastern Pacific coast, expressed in °C per decade. Horizontal axis is month within the year and vertical axis represents location along the coastline. ( b ) Average change in the yearly frequency of extreme hot days, in days per decade. ( c ) Average change in the yearly frequency of extreme cold days, in days per decade. ( d ) Average change in the occurrence of seasonal warming, in days per decade. In b , c and d , significant data are depicted in black and nonsignificant in grey. Numbered black and white portions of the horizontal axis can be used to locate sections of the coastline in the geographical map. Confidence intervals represent s.e.m. Full size image In the Northwest Pacific, from the Bering Strait to the Southwest Sea of Japan, coastal SST has risen at 0.24±0.11 °C per decade, on average. Summer–autumn warming rates have been much higher, however (exceeding 1.0 °C per decade in Northeast Sea of Okhotsk, areas 2–3 in Fig. 6a ), concurrent with increases in the frequency of hot extremes (mean of 13.0±7.3 additional extreme hot days per decade, Fig. 6b ). Also in this area, seasonal warming has been occurring ∼ 6.5 days earlier in the year per decade ( Fig. 6d ). At the same time, some restricted portions of the Kamchatka Peninsula have been witnessing slightly cooler winters and significant increases in the frequency of extreme cold days ( Fig. 6c ). In agreement with previous studies [7] , we also found dramatic increases in temperature further south, along the coasts of the West, Yellow, Eastern China and South China Seas (where rates of 0.5 °C per decade have been exceeded, see Fig. 2a ). There, warming has been occurring mainly in the beginning of the year (reaching ∼ 1.0 °C per decade between January and June, depending on the location, see Fig. 6a ). A marked decrease in the number of extreme cold days was observed southwards from Eastern China Sea (in many locations exceeding 10 days per decade), in association with an increase in the number of extreme hot days ( Fig. 6c and b ). Recent studies suggest that warming off Eastern China is related to large-scale changes in atmospheric and oceanic circulation in the Western Pacific [39] , [40] . Southward from the Southern China Sea (areas 7–13, Fig. 6 ), warming has been homogeneous throughout the year, at a rate of 0.15±0.07 °C per decade. This warming was accompanied by both an increase in the frequency of extreme hot days (5.3±6.3 days per decade in average, Fig. 6b ) and a decrease in extreme cold days (in average, less 9.25±5.71 days per decade, Fig. 6c ). Off Southeast Australia, SST increases, ∼ 0.4 °C per decade, have probably been related to changes in the East Australian Current [41] . Recent reports have shown little changes in the biogeography of coastal species in the region [42] , [43] . 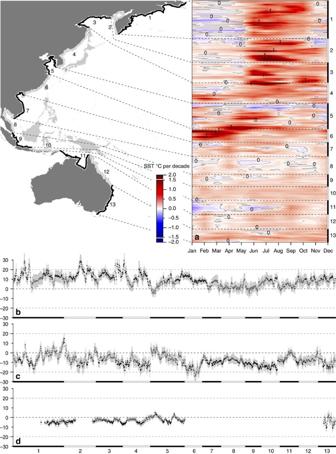Figure 6: Latitudinal transect along the Western Pacific Ocean. (a) Linear trends of SST change along the Western Pacific coast, expressed in °C per decade. Horizontal axis is month within the year and vertical axis represents location along the coastline. (b) Average change in the yearly frequency of extreme hot days, in days per decade. (c) Average change in the yearly frequency of extreme cold days, in days per decade. (d) Average change in the occurrence of seasonal warming, in days per decade. Inb,candd, significant data are depicted in black and nonsignificant in grey. Numbered black and white portions of the horizontal axis can be used to locate sections of the coastline in the geographical map. Confidence intervals represent s.e.m. Figure 6: Latitudinal transect along the Western Pacific Ocean. ( a ) Linear trends of SST change along the Western Pacific coast, expressed in °C per decade. Horizontal axis is month within the year and vertical axis represents location along the coastline. ( b ) Average change in the yearly frequency of extreme hot days, in days per decade. ( c ) Average change in the yearly frequency of extreme cold days, in days per decade. ( d ) Average change in the occurrence of seasonal warming, in days per decade. In b , c and d , significant data are depicted in black and nonsignificant in grey. Numbered black and white portions of the horizontal axis can be used to locate sections of the coastline in the geographical map. Confidence intervals represent s.e.m. Full size image In agreement with other studies [7] , [44] , our assessments of warming along the Eastern Indian Ocean indicated slow continental-scale rates of change. Coastal temperatures have warmed at a mean rate of 0.11±0.09 °C per decade ( Fig. 7a ). Similarly, the frequency of extreme hot days has increased at a relatively slow rate of 4.5±6.8 days per decade ( Fig. 7b ). The frequency of yearly extreme cold days has diminished more rapidly on the coasts of the Bay of Bengal and Andaman Sea, and off Western Sumatra and Southwest Australia (frequently exceeding 10 days per decade, Fig. 7c ). On average, the Northwest and Western coasts of Australia have become colder, especially during austral winter (approximately −1 °C per decade in July off Shark Bay, area 7, Fig. 7 ). A significant increase in the number of extreme cold days was also observed in that region (15 days per decade, Fig. 7c ). The highest warming rates in the Eastern Indian Ocean were observed along the South portion of Australia, especially in the region of the Spencer Gulf, where the warming was matched by a significant increase in the number of extreme hot days and a significant advance of the timing of the seasonal warming ( Fig. 7b,d ). 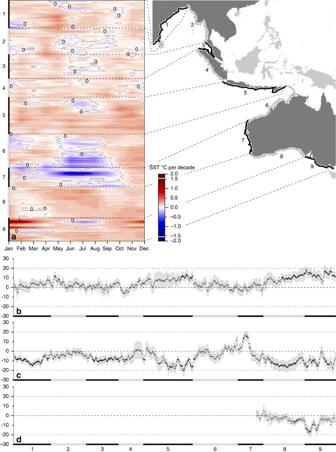Figure 7: Latitudinal transect along the Eastern Indian Ocean. (a) Linear trends of SST change along the Eastern Indian coast, expressed in °C per decade. Horizontal axis is month within the year and vertical axis represents location along the coastline. (b) Average change in the yearly frequency of extreme hot days, in days per decade. (c) Average change in the yearly frequency of extreme cold days, in days per decade. (d) Average change in the occurrence of seasonal warming, in days per decade. Inb,candd, significant data are depicted in black and nonsignificant in grey. Numbered black and white portions of the horizontal axis can be used to locate sections of the coastline in the geographical map. Confidence intervals represent s.e.m. Figure 7: Latitudinal transect along the Eastern Indian Ocean. ( a ) Linear trends of SST change along the Eastern Indian coast, expressed in °C per decade. Horizontal axis is month within the year and vertical axis represents location along the coastline. ( b ) Average change in the yearly frequency of extreme hot days, in days per decade. ( c ) Average change in the yearly frequency of extreme cold days, in days per decade. ( d ) Average change in the occurrence of seasonal warming, in days per decade. In b , c and d , significant data are depicted in black and nonsignificant in grey. Numbered black and white portions of the horizontal axis can be used to locate sections of the coastline in the geographical map. Confidence intervals represent s.e.m. Full size image Coastal SST trends in the Western Indian Ocean were also characterized by moderate changes, although stronger than in the Eastern Indian Ocean (0.18±0.08 °C per decade, Fig. 8a ). The highest temperature increases were observed off Northeast Oman (area 3, Fig. 8a , exceeding ∼ 0.6 °C per decade in April). The Northeast Somali coast has been showing a tendency for colder SSTs during June–August (approximately −0.5 °C per decade, area 4, Fig. 8a ). This coincides with the timing of the Summer Monsoon, when Ekman transport brings upwelled, cooler waters along the coast [23] . The increase in the number of extreme hot days was relatively constant over most of the Western Indian Ocean (6.7±5.4 days per decade on average). Highest increases were observed off Northwest India, between South Yemen and Southeast Tanzania, and along the coast of Southeast Mozambique and Southeast South-Africa ( Fig. 8b ). The yearly frequency of extreme cold days significantly decreased along most of the Western Indian Ocean (at a mean rate of −11.2±6.8 days per decade, Fig. 8c ), the only exception being the relatively small portion of coastline in Northeast Somalia. Off Southeast South-Africa, seasonal warming has been relatively stable (−4.1±4.4 days per decade, see Fig. 8d ). 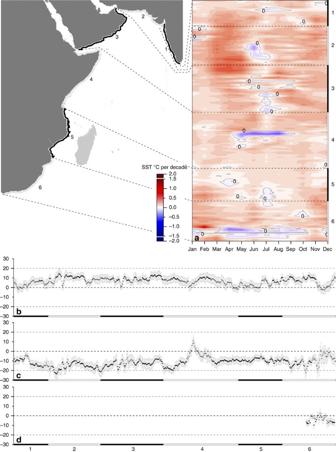Figure 8: Latitudinal transect along the Western Indian Ocean. (a) Linear trends of SST change along the Western Indian coast, expressed in °C per decade. Horizontal axis is month within the year and vertical axis represents location along the coastline. (b) Average change in the yearly frequency of extreme hot days, in days per decade. (c) Average change in the yearly frequency of extreme cold days, in days per decade. (d) Average change in the occurrence of seasonal warming, in days per decade. Inb,candd, significant data are depicted in black and nonsignificant in grey. Numbered black and white portions of the horizontal axis can be used to locate sections of the coastline in the geographical map. Confidence intervals represent s.e.m. Figure 8: Latitudinal transect along the Western Indian Ocean. ( a ) Linear trends of SST change along the Western Indian coast, expressed in °C per decade. Horizontal axis is month within the year and vertical axis represents location along the coastline. ( b ) Average change in the yearly frequency of extreme hot days, in days per decade. ( c ) Average change in the yearly frequency of extreme cold days, in days per decade. ( d ) Average change in the occurrence of seasonal warming, in days per decade. In b , c and d , significant data are depicted in black and nonsignificant in grey. Numbered black and white portions of the horizontal axis can be used to locate sections of the coastline in the geographical map. Confidence intervals represent s.e.m. Full size image When compared with estimates for the global ocean, our study yields higher decadal rates of SST change at the coast. For example, a recent analysis for the period 1960–2009 using HadISST1.1 data reported an oceanic SST rate of change of 0.07 °C per decade and an average change in seasonal timing of −2.3 days per decade [8] . If we also include nonsignificant shifts in our average calculations to make the studies comparable, then our estimates are of 0.18±0.16 °C per decade for SST and −3.3±4.4 days per decade for the seasonal shift. At least partially, these differences might be attributed to the fact that our estimates are based on the last three decades, the period of strongest global warming [5] , [6] . For example, Rayner et al . 's [45] global SST warming rates, using HadSST2, vary from 0.07±0.02 °C per decade to 0.13±0.05 °C per decade when the analysed period changes from 1901–2005 to 1975–2005 (refs 5 and 45 ). Still, it is not surprising that our estimates are closer to the warming rates assessed for the combination of land and ocean ( ∼ 0.2 °C per decade [46] for the last 30 years or 0.16±0.05 °C per decade between 1975 and 2005 (ref. 47 )), given that our analysis was restricted to the oceanic portions closer to land and excluded vast oceanic regions off the continental shelf that have been warming relatively slowly (offshore Pacific, Indian or Southern Oceans) [5] , [6] , [8] . Thus, this study reinforces the notion that coastal systems are among the marine ecosystems most exposed to recent increases in temperature [2] , [7] , which may affect their biodiversity and capacity in delivering important ecosystem services [1] . This study allowed us, for the first time, to analyse the temporal evolution of fine-scale SST patterns in light of broader-scale, global trends. The simultaneously wide and focused perspective is extremely important for studying biogeographic, phenological or community responses to climate change and can also help policy makers and coastal managers make better informed decisions [48] . Our results reveal that even though most coastal areas have been warming worldwide, the magnitude of change has been highly heterogeneous in both space and seasonality, consistent with the heterogeneity of SST on coastal scales [49] . Spatially, there were huge differences across hemispheres and oceanic basins, even among areas with similar oceanographic processes. For example, from the five major upwelling regions worldwide [30] , coastal SST has decreased in the areas of the California and the Humboldt currents (off Eastern United States, Chile and Peru), but have increased in the areas of the Canary, Benguela and Somali currents (off Northeast, Southwest and Northeast Africa). Coupled with findings of increases in both hot and cold temperature extremes along approximately one-tenth of the world's coastlines, these data indicate that global warming is far more complex than a monotonic increase of average temperatures. Most locations have also displayed contrasting warming trends as a function of the season (for example, Northwest Pacific coast). The seasonality of SST changes is extremely important because the same species may display different degrees of vulnerability to thermal stress as a function of its life cycle phase [50] . In addition, owing to the prevalence of changes in the timing of seasonal coastal warming, phenological changes driven by current and future warming are likely to increase [51] . This might be problematic because effects in one species often cascade across trophic webs [36] , [52] and thus single-species perturbations often have broader ecological implications. It is undeniable that a more detailed exploration of the relation between the different regional or seasonal warming regimes and the distinct biotic responses is required. Nonetheless, the changes in temperature here described are likely to potentiate range shifts, invasions and consequent ecological disequilibria [53] , and therefore the analysis of temperature alone might offer a valuable tool for forecasting and pinpointing areas of high risk of biodiversity loss. Data assembly NOAA OI ¼ Degree Daily SST Analysis data [9] were acquired from NOAA's National Climatic Data Center at http://www.ncdc.noaa.gov/oa/climate/research/sst/oi-daily.php . AVHRR-only data were used because it is the only daily SST analysis that extends back to 1981/1982 (ref. 54 ). NOAA's OI algorithm adjusts the satellite data relative to 15 days [55] of quality-controlled in situ ship and buoy data from ICOADS [56] , to achieve long-term stability. There is no evidence for yearly or decadal scale difference in OI SST relative to in situ observations over the period 1985 to 2005 ( Fig. 1 in Reynolds et al . [9] ). NOAA's OI ¼ Degree Daily SST outperformed six other ultra-high resolution models, consistently showing smaller bias and root mean squared errors when matched-up with 18 months of daily in situ SST measured at 13 locations along the coasts of Portugal, Spain and France (see Supplementary Table S1 and Seabra et al . [57] for more details). Daily files from 1 January 1982 to 31 December 2010, each containing daily SSTs and associated s.d. values, were imported into R (ref. 58 ) as georefered layers and stacked in chronological order. Data were retrieved separately for each coastal pixel across the entire assemblage of temporal layers, worldwide. Coastal pixels were defined as those closer to land but with <50% of land contamination, which was assessed using full-resolution GSHHS (Global Self-consistent, Hierarchical, High-resolution Shoreline Database) data [59] . For islands smaller than the analysis scale (0.25°), the pixel with the closest centroid was used. Calculation of warming rates All computations were performed in R (ref. 58 ). For each coastal pixel individually, average warming rates were computed as the slope of the linear regression of seasonally detrended SST versus time, and expressed as °C per decade±s.e.m. To account for errors in the SST OI estimates (including random, sampling and bias errors [9] ), regression parameters were estimated using weighted least squares, with weights inversely proportional to the variance of the SST OI (1/SD 2 ). One of the frequent issues when analysing time series data is the temporal autocorrelation, which can substantially understate the standard error of the trend estimate. To account for this problem, the degrees of freedom (d.f.) were adjusted using the Quenouille procedure [60] , in which N effective = N (1− r )/(1+ r ), with N representing the sample size and r the lag-1 autocorrelation coefficient of the residuals of the seasonally detrended time series. In this way N effective was reduced, on average, from 10,592 to 393, making regressions much more conservative. Spatial autocorrelation biases were avoided by performing all statistical analyses separately for each location; the only exceptions were correlations between the warming rates and the rates of change in the number of extreme days and some data validations described below. In these cases, only 1 of each 20 coastal pixels along the coast were used, corresponding approximately to a separation of 5 degrees, which is far beyond the maximum autocorrelation scale of 250 km reported for the OI SST data set [9] . The projected area of each ¼ degree pixel was used to standardize rates of change per unit of area, before reporting average rates of change over regions. Monthly SST changes were calculated in a similar way, but using monthly averages for each location. Changes in the frequency of extreme events For each location separately, 5 and 95 percentiles of standardized anomalies of the raw SST (1982–2010) were used to define extremely low and extremely high temperature thresholds. Yearly frequencies of daily anomalies exceeding the threshold values were calculated and regressed against time. The Quenouille procedure [60] (see above) was used to correct the degrees of freedom whenever temporal autocorrelation was significant. Regression slopes were then expressed as the average change in the number of days per decade±s.e.m. Changes in the timing of seasonal warming This analysis was restricted to temperate latitudes between 60°S and 30°S, and 30°N and 60°N. For each pixel, the first Julian day in each year exceeding the 75th percentile of the entire SST data set for that geographic location was recorded. For situations in which the Julian date of the first 75th percentile temperature occurred before 1 January (common situation in the southern hemisphere), it was necessary to transform the Julian dates to values <0 to avoid spurious discontinuities in dates associated with the end of the year (for example, if the first day over the 75th SST percentile was 28 December in one year and 2 January in the next, the change in timing was 5 days, not 360). These values were then regressed against time, and slopes expressed as the average change in date per decade±s.e.m. The Quenouille procedure [60] (see above) was used to correct the degrees of freedom when temporal autocorrelation was significant. Controlling for land contamination The requirement for using data from pixels as close as possible to land (so that such pixels would truly represent coastal ecosystems) meant that data could be land contaminated, especially when considering the spatial resolution of NOAA's OI SST data—¼ degree (corresponding approximately to 27.7×24.1 km at 30° latitude and 27.8×13.9 km at 60° latitude). First, this potential problem was mitigated by excluding all pixels overlapping more than 50% with land (as defined by the full-resolution GSHHS coastline data [59] ). Discarding highly land-contaminated pixels decreased the average land fraction from 33.6 to 15.4%. Second, for every coastal pixel (now with a land-overlapping fraction from 0 to 50%), we found the nearest offshore pixel that was completely land-free—see Supplementary Fig. S1a for an example. SST rates of change were then computed for offshore locations, using the same methodology used for coastal pixels. Finally, differences between the warming rates were calculated for each pair of coastal-offshore pixels. If land contamination was significant, one would expect large differences to arise as sampling was moved from coastal to offshore locations. One would also expect differences to be proportional to the percentage of initial land contamination. Instead, the two data sets were highly correlated (Pearson's r =0.99, d.f.=964, P <0.01), diverging only by a small root mean square error—(0.26 °C per decade) and bias (0.04 °C per decade). The difference in temperature between offshore and adjacent land-contaminated pixels was not greater than the difference between offshore and adjacent land-free coastal pixels calculated on pairs of pixels ∼ 500 km apart (two sample t -test, t =0.1242, d.f.=764, P =0.90, see Supplementary Fig. S1b ). More importantly, differences between coastal and offshore pixels were unaffected by the percentage of land contamination displayed by the coastal locations ( Supplementary Fig. S1c ), thereby falsifying the hypothesis that land contamination biased the results. Controlling for long-term changes in cloud contamination NOAA's daily OI data merge day-time and night-time satellite readings into a single SST product. Typically, raw satellite data have a high spatial resolution, but is irregularly spaced due to cloud contamination. Even though the OI process converts these irregularly spaced data into a regular grid, the proportion of daytime and night-time readings used to derive each optimally interpolated pixel will vary on a daily basis due to diel variations in the cloud cover. On the other hand, satellite instruments are only capable of retrieving the temperature of the topmost layer (some microns-thick) of the ocean, which is known to warm by some tenths of degree during the day due to incoming solar radiation [61] , [62] . Therefore, temperatures from daytime readings are typically higher than those obtained during the night. NOAA's OI algorithm adjusts the satellite data relatively to 15 days [55] of quality-controlled in situ ship and buoy data from ICOADS [56] , which greatly reduces the diurnal signal and converts the 'skin' SST to what is known as 'bulk' temperature ( ∼ 0.5 m depth) [9] . Still, it could be argued that a long-term change in the cloud cover or in the diurnal wind cycle would change the long-term balance between the number of individual daytime and night-time measurements contributing to the final interpolated product, and thus affecting the trends assessed in this study. To have a rough estimate of the changes on the diurnal cloud patterns, we selected 18 coastal locations worldwide ( Supplementary Fig. S2 and Supplementary Table S2 ). Selected locations were divided into two groups, based on total cloud (TC) climatology data obtained from the International Satellite Cloud Climatology Project [63] for the period between 1983 and 2009. The first group encompassed locations in areas with historical low levels of cloud cover (41–47%), and the second group included locations in areas usually very cloudy (74–85%). Within each group, locations in open sections and in convoluted stretches of the coast were chosen. Each one of these orthogonal combinations was replicated four times. Separate daytime and night-time AVHRR Pathfinder V5.2 data [64] were obtained for an array of seven by seven 4 km pixels surrounding each one of the 18 coastal locations. Data were obtained through the NOAA's NCDC website at http://pathfinder.nodc.noaa.gov, for the period between 1 January 1982 and 31 December 2010. These data yielded a rough estimate of the number of individual satellite readings contributing to each daily ¼ degree interpolated pixel. The relative proportion of the daytime pixels in relation to night-time pixels was then regressed separately for each location. The Quenouille procedure [60] was used to account for biases due to temporal autocorrelation on the standard errors of the regressions. Results are shown in Supplementary Table S2 : in the 30-year period, there was no evidence for significant changes in the proportion of daytime to night-time satellite data coverage in any of the coastal ¼ degree pixels analysed. This pattern held true irrespective of the cloud climatology or the shape of the coastline (open versus convoluted) associated with each location. How to cite this article: Lima, F. P. & Wethey, D. S. Three decades of high-resolution coastal sea surface temperatures reveal more than warming. Nat. Commun. 3:704 doi: 10.1038/ncomms1713 (2012).